Chemically induced Jahn–Teller ordering on manganite surfaces Physical and electrochemical phenomena at the surfaces of transition metal oxides and their coupling to local functionality remains one of the enigmas of condensed matter physics. Understanding the emergent physical phenomena at surfaces requires the capability to probe the local composition, map order parameter fields and establish their coupling to electronic properties. Here we demonstrate that measuring the sub-30-pm displacements of atoms from high-symmetry positions in the atomically resolved scanning tunnelling microscopy allows the physical order parameter fields to be visualized in real space on the single-atom level. Here, this local crystallographic analysis is applied to the in-situ -grown manganite surfaces. In particular, using direct bond-angle mapping we report direct observation of structural domains on manganite surfaces, and trace their origin to surface-chemistry-induced stabilization of ordered Jahn–Teller displacements. Density functional calculations provide insight into the intriguing interplay between the various degrees of freedom now resolved on the atomic level. Transition metal oxides have emerged as one of the foci for condensed matter physics research due to the multitude of structural, electronic and magnetic phenomena they exhibit [1] , [2] , [3] , opening pathways for multiple device applications [4] and serving as a test bed for development of advanced theoretical models. Many of the same classes of correlated oxides are broadly explored for their electrochemical properties, enabling applications from solid oxide fuel cells to oxygen sensors [5] , [6] , [7] , [8] , and suggesting intrinsic links between physical and electrochemical functionalities. While the bulk properties of these materials are now amenable to a broad range of scattering and electron microscopy techniques, detailed studies of the structure and properties of their surfaces have remained challenging [9] , [10] , [11] , [12] , [13] , [14] . Understanding the emergent physical phenomena at surfaces requires the capability to probe local composition, recognize minute deviations from ideal structures and explore atomic coupling to electronic properties. In this article we report studies of the chemical and electronic structure and structural distortions of the (001) surface of La 5/8 Ca 3/8 MnO 3 (LCMO) through direct mapping by high-resolution scanning tunnelling microscopy (STM), directly visualizing order parameter fields and associated topological defects. The perovskite manganites are a hotbed of exciting physical phenomena enabled by the interplay of structural, electronic and magnetic properties [15] . In addition to unique physical properties, these materials can possess high oxygen non-stoichiometries, affecting their physical behaviours and making them of interest for electrocatalytic applications [16] . Many of these properties are intimately linked to small lattice/angle distortions that can significantly affect their electronic and chemical functionality. From atomic resolution STM images, we identify and refine the surface adatom locations and oxygen vacancies. From these, local distortion angles are extracted based on the refined coordinates of surface adatoms. In this way, we can obtain surface structure maps that clearly demonstrate the boundary between two domains with different distortion orientations. This behaviour is discussed in terms of ordered Jahn–Teller distortions that arise due to the imposed effect of the oxygen adatoms on the surface. Specifically the pattern of oxygen adatoms, that is, the pattern of local oxygen stoichiometry, has a strong influence on the electronic structure of the surface. The surface oxygen adatoms impose a checkerboard pattern of crystal field environments, leading to a charge and orbital disproportionation of the surface Mn lattice. Overall, these studies provide an example of order parameter field mapping from high-resolution STM, opening a pathway for probing electronic properties of topological defects and the interaction between order parameter fields and structural defects. Localization of atomic positions in subpixel precision The (001)-oriented LCMO epitaxial thin films were grown and imaged using STM in-situ under ultra high vacuum. To quantitatively analyse the surface structure and extract order parameter fields from the STM images, we employ a local crystallographic analysis technique extended from the approach originally developed for (scanning) transmission electron microscopy [17] , [18] , [19] , [20] , [21] . Shown in Fig. 1a is a typical STM occupied-state image of a LCMO (√2 × √2)R45° surface area with O adatoms (bright spots) and O vacancies (dark spots), which were studied in detail previously [22] . The origin of the (√2 × √2)R45° on the LCMO surface is different from the √2 × √2 charge-ordering phase on Bi 1− x Ca x MnO 3 surface [9] , and is instead the formation of alternate MnO 6 octahedra (O adatoms) and MnO 5 square pyramids as discussed below. For a quantitative analysis of the structure, we need accurate coordinates of all adatoms and vacancies at the surface. The adatoms are directly visible from the STM images. To visualize the vacancies, we construct a vacancy map using the following procedure. The image is Fourier transformed to provide a 2D reciprocal space pattern. The inverse Fourier transform of the filtered data yields the ideal lattice with full periodicity. By subtracting the ideal lattice from the experimental data in Fig. 1a , a vacancy map, Fig. 1b , is obtained. The initial approximate positions of adatoms ( Fig. 1a ) and vacancies ( Fig. 1b ) can be found using a regular thresholding procedure. We fit two-dimensional Gaussian functions to these approximate positions (170 and 70 pixels per adatom for Fig. 2a and Fig. 2d ) to determine the precise position of each adatom (or ‘false’ atom in a vacancy map) so as to refine the real coordinates of adatoms (or vacancies). This procedure is run iteratively to refine all atoms. Shown in Fig. 1c is the coordinate map of adatoms in Fig. 1a obtained as described above. The coordinated map of vacancies is also obtained as well ( Supplementary Fig. 1 and Supplementary Note 1 ). 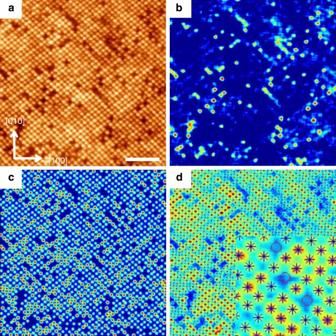Figure 1: Local crystallographic analysis of atomically resolved STM image. (a) Occupied-state STM image of a 20 × 20 nm surface region ofin-situ-grown LCMO film scanned with a bias voltage of −1.75 V (scale bar, 4 nm). (b) Map of oxygen vacancies found using the Fourier filtering procedure. (c) The adatom lattice obtained using the thresholding procedure. (d) Computed locations of adatoms and vacancies overlaid with the topographic image. Calculated locations of adatoms and vacancies are labelled with cross marks and open symbols, respectively. The inset is an expanded map for a better view. Figure 1d shows the superposition of the STM image ( Fig. 1a ) with marks of coordinates of all adatoms ( Fig. 1c ) and vacancies ( Supplementary Fig. 1 ). The marks (cross for adatoms and open circles for vacancies) are overlaid on the topographic image to demonstrate that such a procedure allows for subpixel precision in the localization of atomic positions. Figure 1: Local crystallographic analysis of atomically resolved STM image. ( a ) Occupied-state STM image of a 20 × 20 nm surface region of in-situ -grown LCMO film scanned with a bias voltage of −1.75 V (scale bar, 4 nm). ( b ) Map of oxygen vacancies found using the Fourier filtering procedure. ( c ) The adatom lattice obtained using the thresholding procedure. ( d ) Computed locations of adatoms and vacancies overlaid with the topographic image. Calculated locations of adatoms and vacancies are labelled with cross marks and open symbols, respectively. The inset is an expanded map for a better view. 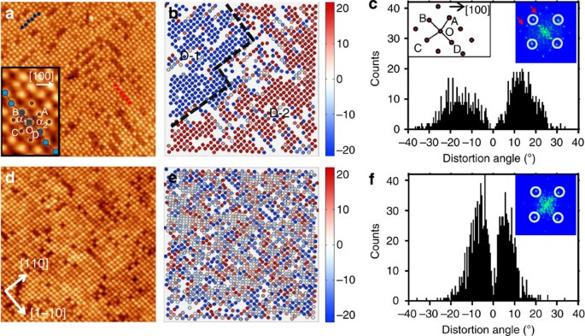Figure 2: Visualizing the distortion domains. (a) Unoccupied-state STM image of LCMO surface with a bias voltage of +1.6 V, 21 × 21 nm. Blue and red circles mark the adatom positions that have zigzag distortions in [110] and [1–10] directions for eye guiding, respectively. An expanded view of the local adatoms with the ABCDO coordinates superimposed is shown in the inset. (b) The distortion angle map of (a) showing two domains with different orientations of distortion angle. See the text for the definition of the sign and value of the angles. The map is plotted such that the colour represents the distortion angle for the adatoms at the locations of the colour spots. Circles are added to better illustrate the locations. (c) Histogram of distortion angles for (a), showing two distinct peaks corresponding to two distortion domains with different orientations. The inset shows the definition of the distortion angles. (d) Occupied-state STM image with a bias voltage of −1.75 V, 20 × 20 nm. (e) The distortion angle map of (d) that does not show any distinct domains comparing with (b). (f) Histogram of distortion angles for (d), showing smaller distortions. The FFT of (a) and (d) are shown in the insets of (c) and (f). Spots in the white circles are from (√2 × √2)R45°; extra spots pointed by red arrows are only shown in the unoccupied-state image, but not in the occupied-state image. Full size image Figure 2: Visualizing the distortion domains. ( a ) Unoccupied-state STM image of LCMO surface with a bias voltage of +1.6 V, 21 × 21 nm. Blue and red circles mark the adatom positions that have zigzag distortions in [110] and [1–10] directions for eye guiding, respectively. An expanded view of the local adatoms with the ABCDO coordinates superimposed is shown in the inset. ( b ) The distortion angle map of ( a ) showing two domains with different orientations of distortion angle. See the text for the definition of the sign and value of the angles. The map is plotted such that the colour represents the distortion angle for the adatoms at the locations of the colour spots. Circles are added to better illustrate the locations. ( c ) Histogram of distortion angles for ( a ), showing two distinct peaks corresponding to two distortion domains with different orientations. The inset shows the definition of the distortion angles. ( d ) Occupied-state STM image with a bias voltage of −1.75 V, 20 × 20 nm. ( e ) The distortion angle map of ( d ) that does not show any distinct domains comparing with ( b ). ( f ) Histogram of distortion angles for ( d ), showing smaller distortions. The FFT of ( a ) and ( d ) are shown in the insets of ( c ) and ( f ). Spots in the white circles are from (√2 × √2)R45°; extra spots pointed by red arrows are only shown in the unoccupied-state image, but not in the occupied-state image. Full size image Visualizing the distortion domains The information on atomic position can be further explored to visualize the ordered structural distortions on the surface. The distortions are not readily obvious in the unoccupied-state topographic image ( Fig. 2a ), but close inspection reveals a zigzag pattern of displacements along either the [1–10] or the [110] directions of the cubic perovskite structure, as highlighted by the red and blue solid circles, respectively. Using the refined atomic positions, the distortion angle map can be analysed quantitatively using the procedure schematized in the inset of Fig. 2c . For each adatom O, we define four vectors to its nearest neighbours: OA, OB, OC and OD, and assign indices defined by the quadrant in which they are located. Subsequently we define α 1 as the angle between OA and OC and α 2 as the angle between OB and OD. To easily visualize the directions of the zigzag, a sign was assigned to the distortion based on the distortion direction. If α 1 is the angle that deviates the most from 180°, a negative distortion angle with magnitude | α 1 –180|° is assigned; if α 2 is the angle that deviates the most from 180°, a positive distortion angle with magnitude | α 2 –180|° is assigned. In this way a distortion map can be constructed with distortions along [110] having different signs from distortions along [1–10]. Figure 2b is the distortion map of Fig. 2a , revealing two distinct distortion domains. In domain D-1, adatoms are alternately shifted towards ±[1–10] directions, forming a zigzag pattern along [110], while in domain D-2, the adatoms are alternately shifted towards ±[110], forming zigzags along [1–10]. The angle distortion map also reveals the boundary between D-1 and D-2, clearly visualizing two structural distortion domains; the black dashed line is added as a guide. The distortion angle histogram ( Fig. 2c ) clearly shows two distinct peaks with different signs, with centres at about ±14°, which corresponds to a 30-pm displacement of atoms from high-symmetry positions in the atomically resolved STM (see Supplementary Fig. 2 and Supplementary Note 2 for more details). The distortion angles are independent of the value of the tip voltage within the unoccupied states. We further explore the surface in terms of the influence of tip polarity on the distortion. Figure 2d shows a topographic image taken at negative bias (occupied states), where ordered zigzag lines are conspicuously absent (see Supplementary Fig. 3 for dual bias images at the same area). The distortion angle map for the image ( Fig. 2e ) does not reveal any distinct distortion domains, most likely because the domains are much smaller combined with the frustration for the distortion pattern at the ubiquitous domain boundaries. The histogram of distortion angles, Fig. 2f , shows peaks very close to zero, which contrasts distinctly with Fig. 2c , see below. Although the 30-pm displacements of atoms from high-symmetry positions is hard to extract from the image directly, Fast Fourier Transforms (FFT) of the images clearly show the extra spots corresponding to the deformation. The insets in Fig. 2c, f show the FFT of the unoccupied- and occupied-state images. Extra spots from the deformation can be seen readily, as indicated by red arrows in the unoccupied-state (positive bias) image but not in the occupied-state (negative bias) image. Local electronic structure of two classes of Mn coordination The zigzag distortions along the [110] and [1–10] directions observed on the surface cannot originate from the bulk. For this composition ( x =3/8) the in-plane cell is √2 a × √2 a , where a is the cubic perovskite lattice parameter [23] . Here, the zigzag pattern expands the surface cell to 2√2 a × √2 a , with the long axis along the zigzag chain, reminiscent of the Jahn–Teller distortions of the charge/orbital order of half-doped LCMO ( x =0.5) (ref. 24 ). To explore the possibility of charge and orbital order, first-principles calculations of the manganite surface were performed in the framework of density functional theory. We modelled the chemical doping of LCMO via the virtual crystal approximation, where we replace La ions in LaMnO 3 with pseudopotentials having non-integer atomic number corresponding to 3/8 holes per formula unit. We restricted the in-plane pseudocubic lattice constant to a =3.937 Å, which is the equilibrium lattice constant for bulk cubic SrTiO 3 (STO) in our DFT calculations, in order to simulate fully coherent epitaxial growth on an STO substrate. Bulk calculations were performed for our model LCMO on a 4 × 4 × 3 k -point mesh using a 20-atom orthorhombic cell, that is, 4 formula units, with in-plane lattice vectors having length √2 a rotated by 45° with respect to the pseudocubic lattice vectors of the substrate. This expansion of the cell was required to take into account tilts and rotations of the oxygen octahedra. The small lattice mismatch with respect to STO results in a bulk pseudocubic c / a ratio of 0.998, consistent with what is known from experiment for many of the hole-doped La-manganites [23] . To study the surface properties, we constructed a supercell with a 10.5 unit-cell thick slab of our model LCMO, terminated on both sides with MnO 2 , and ~40 Å of vacuum separating periodic images along the direction perpendicular to the plane of the slab (see Fig. 3a ). At the surface we placed oxygen adatoms above half of the surface Mn sites, consistent with the (√2 × √2)R45° construction observed by STM [22] . Atomic relaxations for this structure were performed on a 4 × 4 × 1 k -point sampling of the entire Brillouin Zone, followed by a 10 × 10 × 1 static lattice calculation to refine electronic structure. Due to computational limitations, we limited our calculations to the same √2 a × √2 a in-plane cell used for the bulk. While this cell cannot incorporate the Jahn–Teller structural order, we examined the electronic structure to look for the tell-tale signatures of the charge/orbitally ordered state. In addition, all Mn magnetic moments were assumed to be ferromagnetically ordered in the calculation. 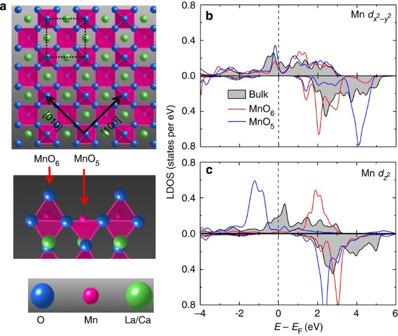Figure 3: Structure model and calculated density of states. (a) Relaxed structure of the LCMO surface (√2 × √2)R45° structure (top view and side view). (b,c) Local density of states (LDOS) projected onto the Mnegorbitals. Filled curves correspond to bulk sites. Red and blue curves correspond to the MnO6and MnO5surface sites, respectively. (b) Projection ontoorbitals. (c) Projection ontoorbitals. The top and bottom panels correspond to the majority and minority spin channels, respectively, and the vertical dashed lines indicate the Fermi level,EF. Figure 3: Structure model and calculated density of states. ( a ) Relaxed structure of the LCMO surface (√2 × √2)R45° structure (top view and side view). ( b , c ) Local density of states (LDOS) projected onto the Mn e g orbitals. Filled curves correspond to bulk sites. Red and blue curves correspond to the MnO 6 and MnO 5 surface sites, respectively. ( b ) Projection onto orbitals. ( c ) Projection onto orbitals. The top and bottom panels correspond to the majority and minority spin channels, respectively, and the vertical dashed lines indicate the Fermi level, E F . Full size image There are two classes of Mn coordination at the surface due to the arrangement of oxygen adatoms: MnO 6 octahedra and MnO 5 square pyramids, as shown in the side view of Fig. 3a . In addition, the MnO 6 octahedra at the surface differ from the bulk MnO 6 in that there is a significant displacement of the Mn from the centre of the octahedron [25] . This arises due to the polar nature of LCMO, consisting of formally charged (001) atomic layers of [(La,Ca)O] 5/8+ and [MnO 2 ] 5/8− (ref. 26 ). The MnO 2 surface is negatively charged, giving rise to an electric field in the LCMO pointing towards the surface, which pushes the Mn upward while pulling the O down [25] . The different crystal field environments on the two types of Mn sites give rise to a significant difference in local electronic structure. This can be seen in Fig. 3b,c , where we plot the local density of states of the Mn e g orbitals ( Fig. 3c ) and ( Fig. 3b ), where z is perpendicular to the surface and x and y correspond to the [100] and [010] directions, respectively. First, we note that the electronic structure in this ferromagnetic state is half-metallic, with a gap in the minority spin channel, consistent with what is expected for the hole-doped manganites. Therefore, we will limit the remainder of our discussion to the majority spin states, where the important physics is contained. Similar to the bulk, both surface Mn sites have partial occupancy of the orbitals, with more weight on the MnO 5 sites ( Fig. 3b ). On the other hand, the occupancy of the channel is disproportionate ( Fig. 3c ): the orbitals on the MnO 6 sites are pushed significantly above the Fermi level, whereas on the MnO 5 sites the states are fully occupied. This disproportionation of the occupancy follows directly from the different environments surrounding the two Mn sites, as illustrated in Fig. 4 . First, a simplistic electron-counting argument reveals that the missing O 2− ion in the MnO 5 sites leaves more electrons on the Mn, and therefore should tend to bias the site toward a d 4 (Mn 3+ ) state, where there should be occupancy of the e g manifold. Second, the absence of an apex O 2− ion on the MnO 5 pyramid significantly lowers the crystal field energy of the orbital with respect to orbitals, which are relatively unperturbed by the presence or absence of an apex O 2− ion (see Fig. 4a ). Furthermore, the off-centring of the Mn ion in the MnO 6 sites increases the crystal field energy of the orbital even more with respect to a centrosymmetric structure, therefore suppressing its occupancy and tending the site towards a d 3 (Mn 4+ ) state ( Fig. 4a ). This kind of ordering of the Mn occupancy is not unlike the spontaneous ordering expected for half-doped LCMO, but in this case it is enforced by the (√2 × √2)R45° ordering of oxygen adatoms. 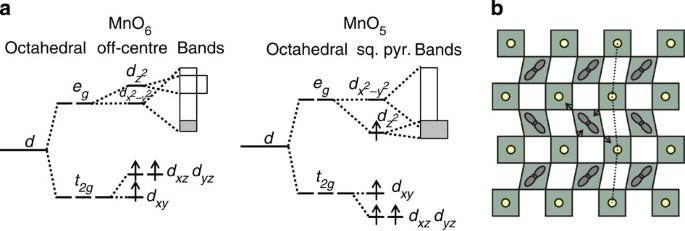Figure 4:The formation of the ordered Jahn–Teller distortions. (a) Crystal field splitting of Mn-dorbitals in MnO6and MnO5sites. The band formation is shown schematically for theegorbitals, where the grey colour indicates occupation. (b) Schematic of the ordered Jahn–Teller distortions on the LCMO surface. Squares represent the MnO6sites, with yellow circles indicating the positions of the oxygen adatoms. Parallelograms represent the distorted MnO5pyramids, with the lower energy orbital schematically shown. The Jahn–Teller distortion on the central site is indicated by arrows. The vertical dashed zigzag indicates the zigzag distortion of oxygen adatoms along [110]. Figure 4: The formation of the ordered Jahn – Teller distortions. ( a ) Crystal field splitting of Mn- d orbitals in MnO 6 and MnO 5 sites. The band formation is shown schematically for the e g orbitals, where the grey colour indicates occupation. ( b ) Schematic of the ordered Jahn–Teller distortions on the LCMO surface. Squares represent the MnO 6 sites, with yellow circles indicating the positions of the oxygen adatoms. Parallelograms represent the distorted MnO 5 pyramids, with the lower energy orbital schematically shown. The Jahn–Teller distortion on the central site is indicated by arrows. The vertical dashed zigzag indicates the zigzag distortion of oxygen adatoms along [110]. Full size image Formation and lift of the Jahn–Teller distortion Given that the MnO 5 sites have both and character, whereas the MnO 6 sites have only character, one expects only the MnO 5 sites to be susceptible to a Jahn–Teller distortion. Occupancy of both and states means that the MnO 5 sites in a square pyramidal geometry have an orbital degeneracy between and states (that is, , respectively). This degeneracy can be lifted by a new Jahn–Teller distortion of the basal plane of the pyramid corresponding to stretching along either the [100] or the [010] axis, and contraction along the other, as shown schematically on the central site in Fig. 4b . The effect on the MnO 6 octahedra is to alternately shift distortions along [1–10], leading to a zigzag pattern of displacements of oxygen adatoms along [110] as observed in the STM data. Only one type of Jahn–Teller domain is shown in Fig. 4b ; the other type corresponds to an in-plane rotation of Fig. 4b by 90°, with a zigzag pattern along [1–10]. Both domains are seen in the STM images ( Fig. 2 ). For a negative tip bias, electrons in the LCMO film will be pushed away from the surface towards the bulk in response to the electric field between the tip and the surface. Looking at Fig. 3b we see that this will lead to at least a partial depletion of the orbitals, and therefore can lead to a diminishing or suppressed Jahn–Teller distortion: non-zero occupancy of both and orbitals is required for energy lowering by symmetry breaking of a square pyramidal crystal field. For positive tip bias, the situation is reversed: electrons will move toward the surface to screen the electric field, and further fill the states, leading perhaps to an enhancement of the Jahn–Teller mechanism. This is consistent with the sharp difference between positive and negative tip bias images ( Fig. 2a,d ). For positive tip bias, the zigzag pattern is apparent, and is consistent with the Jahn–Teller displacement pattern discussed above and shown in Fig. 4b . For negative bias, however, the distortions are reduced in magnitude ( Fig. 2f ) and less ordered ( Fig. 2d ) due to the charging of the surface by the polarity of the tip. Using high-resolution STM imaging with direct structural crystallographic analysis we have achieved direct visualization of the structure of an ordered oxygen adatom array on a complex oxide surface. In particular, we directly observed surface Jahn–Teller domains, which are unexpected for this stoichiometry. This behaviour can be traced directly to the chemical environment of the surface, namely the pattern of oxygen adatoms has a strong influence on the electronic structure of the surface. The surface oxygen adatoms impose a checkerboard pattern of crystal field environments, leading to a charge and orbital disproportionation of the surface Mn lattice. The observed zigzag structural domains are associated with ordered Jahn–Teller distortions on the MnO 5 sites. This study opens a new pathway to explore the interplay between atomic, structural and electronic degrees of freedom on the atomic state, and should afford new opportunities in the study of complex oxide surfaces. Samples The LCMO epitaxial thin films were grown on Nb-doped STO single-crystal substrates using laser molecular beam epitaxy (laser MBE) [22] . The Nb-doped STO substrates were chemically etched by buffered HF followed by ex-situ annealing in a flowing oxygen environment at 950 °C and in-situ annealing at 820 °C for 30 min to ensure a well-ordered TiO 2 terminated surface [27] . The growth was carried out in an ultra-high vacuum system with a base pressure of 3 × 10 −10 Torr as reported elsewhere [22] . During growth, the substrate was kept at about 820 °C in a flowing oxygen (8% ozone) environment under a pressure of 7 × 10 −4 Torr. Differentially pumped reflection high-energy electron diffraction was used to monitor the growth quality. After growth, samples with a film thickness of 120 nm were annealed in situ at 820 °C for 30 min and then allowed to cool under the same oxygen pressure as that of growth. After cooling, oxygen was pumped out and samples were immediately transferred in situ to a STM chamber with a base pressure of 1 × 10 −10 Torr. Surface morphology All STM images were acquired at a pressure of 1 × 10 −10 Torr using mechanically cut Pt–Ir tips. In our configuration, a positive or a negative bias image reveals unoccupied or occupied local density states of the sample surface, respectively. Calculation First-principles calculations of the manganite surface were performed in the framework of density functional theory calculations of the manganite surface using the pseudopotential plane-wave code QuantumESPRESSO [28] . The Perdew–Burke–Ernzerhof generalized gradient approximation was employed as the density functional [29] , and plane-wave expansions of the wave functions employed a cutoff of 400 eV. How to cite this article: Gai, Z. et al . Chemically induced Jahn–Teller ordering on manganite surfaces. Nat. Commun. 5:4528 doi: 10.1038/ncomms5528 (2014).